Molecular reorientation of a nematic liquid crystal by thermal expansion A unique feature of nematic liquid crystals is orientational order of molecules that can be controlled by electromagnetic fields, surface modifications and pressure gradients. Here we demonstrate a new effect in which the orientation of nematic liquid crystal molecules is altered by thermal expansion. Thermal expansion (or contraction) causes the nematic liquid crystal to flow; the flow imposes a realigning torque on the nematic liquid crystal molecules and the optic axis. The optical and mechanical responses activated by a simple temperature change can be used in sensing, photonics, microfluidic, optofluidic and lab-on-a-chip applications as they do not require externally imposed gradients of temperature, pressure, surface realignment, nor electromagnetic fields. The effect has important ramifications for the current search of the biaxial nematic phase as the optical features of thermally induced structural changes in the uniaxial nematic liquid crystal mimic the features expected of the biaxial nematic liquid crystal. Materials expand when heated and contract when cooled because of temperature-induced changes in distances between molecules and atoms. Thermal expansion does not change overall structure of the material. Expanding mercury in a thermometer remains an isotropic fluid and an expanding crystal preserves its crystallographic symmetry. In this work, we demonstrate that thermal expansion and contraction of a uniaxial nematic liquid crystal (NLC), an intermediate state of matter between an isotropic fluid and a solid crystal with a long-range orientational order but no long-range positional order, does change the structure by realigning the constituent molecules. Liquid crystals (LCs) are finding numerous applications because of their ability to change orientation of molecules in response to very weak physical and chemical cues, such as electromagnetic fields, surface modifications and pressure gradients. In the uniaxial NLC, the preferred orientation of molecules, the so-called director n̂ , is also the local optic axis associated with a significant optical anisotropy (birefringence and dichroism). Reorientation of the optic axis n̂ is used in information displays [1] driven by the electric field, biomedical and chemical sensing based on surface interactions [2] , [3] , [4] , in microfluidic and optofluidic devices controlled by pressure gradients [5] , [6] , [7] . In the description of dynamic response of NLC to the external fields, boundary conditions and their gradients, it is assumed that the NLC density and volume are constant, independent of molecular reorientation and materials flow [8] . This 'incompressible flow' assumption is a natural extension of a similar simplification in the hydrodynamics of isotropic fluids [9] . The simplification is well justified when the velocities of interest are slower than the speed of sound. However, when the fluid is heated or cooled, it expands or shrinks. The change of volume must be accompanied by flow, because of the mass conservation principle. Surprisingly, even for the isotropic fluids, this thermo-mechanical effect has not been pursued in the literature until 2004, when Yariv and Brenner [10] explored how an unsteady temperature field causes a flow of an isotropic fluid. Tripathi et al . [11] extended the consideration to describe microfluidic DNA amplification in rectangular capillaries. Braun et al . [12] used a focused laser beam as a heat source of thermal waves that drive microflows of isotropic fluids. In this work, we demonstrate that volume changes during heating and cooling of NLC samples generate flows that cause pronounced reorientation of molecules and of the optic axis n̂ . For the NLC in a long rectangular capillary with open ends, we establish the flow velocity dependence on the distance from the centre of the sample and determine the flow-induced distortions of n̂ in the vertical cross section of the capillary, using 3D optical microscopy. Under the action of the flow-induced shear, the director tilts in two opposite directions in the top and the bottom parts of the capillary. The director tilts cause dramatic changes of the optical appearance of the uniaxial NLC sample. In the transient flow-induced state, the uniaxial NLC sample mimics optical features expected of the biaxial NLC. We show that the expansion/contraction flows can be used for transport of colloidal particles in the NLC. We propose an analytical model that explains the flow, director tilt and optical features as a result of thermal expansion/contraction. The effect is general for many different NLC materials, both thermotropic and lyotropic (solvent-based) and represents a new powerful tool to control optical properties of NLCs and transport of particles in them. The ability to realign the optic axis by the changing temperature fields offers numerous applications in sensing, microfluidic, optofluidic, lab-on-a-chip devices. It allows one to build devices with a very simple design as no pressure pumps are needed to generate flow and realign molecules. Behaviour of NLCs in capillary The simplest geometry to observe and characterize the new thermo-optical effect is to place a typical NLC, such as the mixture E7 (EM Industries), in a rectangular long quartz capillary that orients n̂ perpendicularly to the top and bottom flat boundaries, along the vertical z axis, Fig. 1 (the so-called homeotropic alignment). The ends of capillary are open. The capillary thickness d =50 μm (measured along the z axis) is much smaller than its width 1 mm (along the y axis) and length 5 cm (along the x axis) ( Fig. 1a ). At the lateral edges of the capillary and in the meniscus regions near the open ends, n̂ deviates from the vertical z axis; however, extension of these distortions is only a few tens of micrometres and it does not affect much the perfect homeotropic area of size 1 mm×5 cm. In what follows, we describe the properties of the initial homeotropic area, away from the distorted edges. 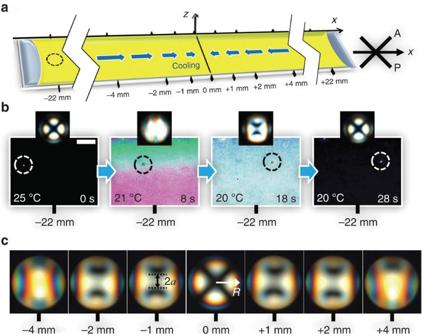Figure 1: Optical response and dynamics of colloidal particles. (a) Capillary of thicknessd=50 μm filled with E7 and fluorescent particles. (b) Time sequence of polarizing microscopy textures at the locationx=−22 mm (marked by a circle in panela), when the sample is cooled from 25 to 20 °C with the rateξ=−30 °C min−1. The texture changes from dark at constantT=25 °C to bright because of the NLC flow (as seen by following the particle marked by a circle) that tilts the director. As the temperature stabilizes at 20 °C, the bright birefringent texture relaxes back to the dark texture of a uniform homeotropic NLC. The insets show the time evolution of the corresponding conoscopic textures at the same locationx=−22 mm. Scale bar is 50 μm. (c) Conoscopic textures of different locations alongx. At fixedT, the textures represent a Maltese cross characteristic of a homeotropic uniaxial NLC. AsTvaries from 25 to 20 °C (ξ=−30 °C min−1), the isogyres split; the split distance 2aincreases with the distance |x| from the capillary center. The movie version of (b) is available in theSupplementary Information(Supplementary Movie 1). Figure 1: Optical response and dynamics of colloidal particles. ( a ) Capillary of thickness d =50 μm filled with E7 and fluorescent particles. ( b ) Time sequence of polarizing microscopy textures at the location x =−22 mm (marked by a circle in panel a ), when the sample is cooled from 25 to 20 °C with the rate ξ =−30 °C min −1 . The texture changes from dark at constant T =25 °C to bright because of the NLC flow (as seen by following the particle marked by a circle) that tilts the director. As the temperature stabilizes at 20 °C, the bright birefringent texture relaxes back to the dark texture of a uniform homeotropic NLC. The insets show the time evolution of the corresponding conoscopic textures at the same location x =−22 mm. Scale bar is 50 μm. ( c ) Conoscopic textures of different locations along x . At fixed T , the textures represent a Maltese cross characteristic of a homeotropic uniaxial NLC. As T varies from 25 to 20 °C ( ξ =−30 °C min −1 ), the isogyres split; the split distance 2 a increases with the distance | x | from the capillary center. The movie version of ( b ) is available in the Supplementary Information ( Supplementary Movie 1 ). Full size image The optical appearance of the homeotropic NLC viewed between two crossed polarizers of an optical polarizing microscope (PM) is very different when the temperature T is fixed and when it is changing ( Fig. 1b ). When T =const, the texture is dark ( Fig. 1b ) as the optic axis n̂ is along the direction z of light propagation. Once the temperature starts to change, the texture brightens ( Fig. 1b and Supplementary Movie 1 ). The bright appearance is caused by the director tilt away from the z axis and toward the expansion direction (the x axis), as established by conoscopic observations, with the sample illuminated by a converging cone of light [13] . The conoscopic texture of the initial homeotropic state represents a symmetric Maltese cross (the two end insets in Fig. 1b ). When the temperature changes, the cross splits into two isogyres, indicating that n̂ tilts to the left and to the right from the vertical z axis, remaining within the x, z plane [14] . The splitting of isogyres (and thus the tilt of n̂ ) increases with the distance | x | from the capillary center ( Fig. 1c ). The director tilt is associated with the material flow, as visualized by fluorescent latex spheres of diameter 2 μm added to the NLC ( Fig. 1b ). Following trajectories of the particles, we determined the maximum flow velocity v x during the temperature change, as a function of horizontal coordinate x , for different initial temperatures T ( t =0)= T 0 of the sample, but fixed increment Δ T = T − T 0 , and change rate ξ = ∂T / ∂t =±30 °C min −1 . The velocity v x is proportional to x and increases as T 0 decreases ( Fig. 2a,b ). The transient dynamics of NLC depends on T 0 , Δ T , ξ and sample thickness d . In particular, for E7 with T 0 =25 °C, Δ T =−5 °C, ξ =−30 °C min −1 , d =50 μm, the bright texture persists for 25 s. To characterize the flow relaxation, we measured the time interval t r between the start of temperature change, t =0, and the time t r when the dispersed particles stopped to move. This relaxation time increases with |Δ T |, | ξ | and d and decreases at higher T 0 ; a typical dependence t r ( d , T 0 ) is shown in Fig. 2c . At low temperatures and in thick samples, t r can be in the range of many minutes and even hours. 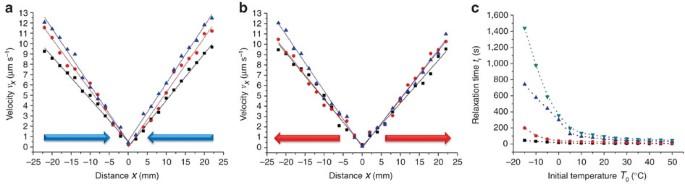Figure 2: Flow velocity and decay time. (a) Maximum flow velocity as a function of coordinatexalong the capillary axis in the regime of cooling (SquareT0=25 °C, circleT0=15 °C, triangleT0=5 °C, ΔT=−5 °C and ξ=−30 °C min−1). (b), The same for heating (SquareT0=20 °C, circleT0=10 °C, triangleT0=0 °C, ΔT=+5 °C and ξ=+30 °C min−1); capillary of thicknessd=50 μm filled with E7. (c) Relaxation timetras the function of cell thickness and the initial temperatureT0of the homeotropic E7 cell (Squared=20 μm, circled=50 μm, up-pointing triangled=100 μm, down-pointing triangled=200 μm);T=−5 °C;ξ=−30 °C min−1. Figure 2: Flow velocity and decay time. ( a ) Maximum flow velocity as a function of coordinate x along the capillary axis in the regime of cooling (Square T 0 =25 °C, circle T 0 =15 °C, triangle T 0 =5 °C, Δ T =−5 °C and ξ=−30 °C min −1 ). ( b ), The same for heating (Square T 0 =20 °C, circle T 0 =10 °C, triangle T 0 =0 °C, Δ T =+5 °C and ξ=+30 °C min −1 ); capillary of thickness d =50 μm filled with E7. ( c ) Relaxation time t r as the function of cell thickness and the initial temperature T 0 of the homeotropic E7 cell (Square d =20 μm, circle d =50 μm, up-pointing triangle d =100 μm, down-pointing triangle d =200 μm); T =−5 °C; ξ =−30 °C min −1 . Full size image Director profile in shear ( xz ) plane To elucidate the link between the director tilt and the material flow, we used fluorescent confocal polarizing microscopy (FCPM) to map the director profile as a function of time and all three spatial coordinates [15] . Of especial interest is the director distortion in the shear ( xz ) plane ( Fig. 1a ). The resolution of 3D images of the director profile is greatly improved when birefringence of the NLC is low [15] . Because of this, we performed experiments not only with highly birefringent E7 but also with the nematic MLC-6815 (EM Industries) of low birefringence, doped with an anisometric fluorescent dye. The sample is probed by a linearly polarized laser beam that causes the dye to fluoresce. The intensity of fluorescence I FCPM depends on the angle α between the polarization P of the beam and n̂ : I FCPM ∞ cos 4 α (ref. 15 ). The optical scan of the sample in the vertical plane ( xz ) ( Fig. 3a,b ) allows us to extract the data on I FCPM ( x, z ) ( Fig. 3c,d ) and thus n̂ ( Fig. 3e,f ). 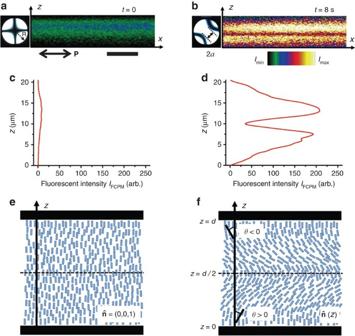Figure 3: Director configurations in the vertical cross-section of the NLC cell. (a) FCPM texture of the vertical cross-section (xz) of a homeotropic cell of thicknessd=20 μm filled with MCL-6815; the probing laser beam is polarized along the directionP; scale bar is 20 μm. The inset on the left-hand side shows a conoscopic Maltese cross. The temperature is fixed at −15 °C. (b) FCPM texture of the vertical cross-section (xz) of the same cell, during cooling from −15 to −25 °C, with the rateξ=−30 °C min−1. (c) The fluorescence signal intensity as a function of the vertical coordinatezfor the initial state. (d) The same for the thermally contracted state; thez-dependence of the FCPM signal show two pronounced maxima and three minima, near the bounding plates and in the middle plane. (e) The reconstructed director profile in the homeotropic state at fixedT=−15 °C. (f) The reconstructed bow-shaped director profile in the cooling-induced tilted state att=8 s. Figure 3: Director configurations in the vertical cross-section of the NLC cell. ( a ) FCPM texture of the vertical cross-section ( xz ) of a homeotropic cell of thickness d =20 μm filled with MCL-6815; the probing laser beam is polarized along the direction P ; scale bar is 20 μm. The inset on the left-hand side shows a conoscopic Maltese cross. The temperature is fixed at −15 °C. ( b ) FCPM texture of the vertical cross-section ( xz ) of the same cell, during cooling from −15 to −25 °C, with the rate ξ =−30 °C min −1 . ( c ) The fluorescence signal intensity as a function of the vertical coordinate z for the initial state. ( d ) The same for the thermally contracted state; the z -dependence of the FCPM signal show two pronounced maxima and three minima, near the bounding plates and in the middle plane. ( e ) The reconstructed director profile in the homeotropic state at fixed T =−15 °C. ( f ) The reconstructed bow-shaped director profile in the cooling-induced tilted state at t =8 s. Full size image At fixed temperature, I FCPM ( x , z ) is close to zero, as n̂ is perpendicular to P ( Fig. 3a,c,e ). A small background signal in Fig. 3a,c is due to director fluctuations. When the temperature changes, the fluorescent intensity I FCPM ( z ) profile shows two well-resolved maxima ( Fig. 3b,d ). It implies that n̂ remains vertical at the cell's boundaries z =0, d , and in the middle plane, z = d /2, but tilts into two opposite directions in the top and bottom parts of the cell, forming a bow-type structure ( Fig. 3f ). The maximum director tilt θ measured with respect to the z axis is about 20°. The non-uniform director profile along the z axis explains the bright birefringent textures ( Fig. 1b ) and splitting of isogyres shown in Fig. 1c and also in the left-hand side inset in Fig. 3b . As the temperature stabilizes, the NLC relaxes back to the initial homeotropic state. 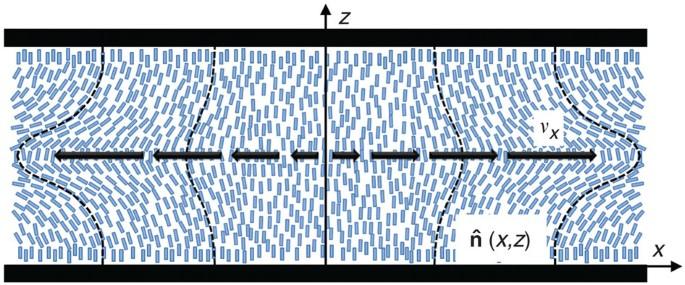Figure 4: Horizontal flow velocity and director configuration. Vertical cross-section of a capillary filled with a thermally expanding NLC, as a function of horizontal coordinatexand vertical coordinatez. Figure 4 summarizes schematically the experimental data on the horizontal velocity and flow-induced director distortions in the thermally expanding NLC. The velocity and director field are shown for the vertical cross-section ( x,z ) of the capillary, which is also the shear plane. Figure 4: Horizontal flow velocity and director configuration. Vertical cross-section of a capillary filled with a thermally expanding NLC, as a function of horizontal coordinate x and vertical coordinate z . Full size image The homeotropic-to-bow-state transition just established is similar to the one observed in refs 16 , 17 , 18 , 19 , 20 , with that difference that in the prior works, the textural transformations were created by the pressure-driven Poiseuille flows, whereas in this work the effect results from thermal expansion; there are no pumps. Note that possible temperature gradients are not the cause of the observed effect ( Supplementary Method ), although they can be certainly added to the list of control parameters if desired. Other types of LCs and geometries The thermally induced director realignment described above and summarized in Fig. 4 refers to an initially uniform thermotropic NLC. In the Supplementary Fig. S1 , we demonstrate that the same phenomenon can be staged in many other NLCs, such as the thermotropic liquid crystal pentylcyanobiphenyl (5CB), mixtures MLC-6815 and ZLI-2806 and the lyotropic NLC Sunset Yellow. At a fixed temperature, conoscopy textures of homeotropic samples of all these materials show a stable dark Maltese cross (first column in Supplementary Fig. S1 ). As the temperature varies, the cross splits into two symmetric isogyres indicating the tilt of n̂ (middle column in Supplementary Fig. S1 ). After a certain relaxation time, the split isogyers relax back to the initial Maltese cross (right column in Supplementary Fig. S1 ). Supplementary Figure S2 and Supplementary Movie 2 show the thermally induced reorientation of molecules in a tangentially anchored cells ( n̂ is in the plane of cells, but there is no preferred orientation in that plane). The sample contains linear defects disclinations [21] around which n̂ reorients by 180°. The disclinations are topologically stable as there is no continuous deformation of the director field that can transform them into a uniform director state. The ends of each disclination are located at the opposite plates. If the temperature is fixed, the disclinations are more or less parallel to the vertical axis z to minimize the energy of elastic distortions ( Supplementary Fig. S2a) . As the temperature is changed to generate NLC flow, the disclinations are stretched in the direction of flow, but their ends remain pinned at the surface irregularities ( Supplementary Fig. S2b and Supplementary Movie 2 ). The stretching of disclinations in the thermally activated NLC can be used for controlled in-plane switching of the optical axis, as n̂ rotates by 90° in going from one side of the disclination to the other ( Supplementary Fig. S2a (inset)). Supplementary Figure S3 shows the molecular reorientation by thermally induced flow in a homogeneous planar cell, with n̂ parallel to a single direction in the plane of the cell. To achieve the planar anchoring, we spin-coated polyimide PI-2555 (Dupont) onto the glass substrates and then rubbed it unidirectionally. The cell was filled with E7 doped with the anisometric fluorescent dye N , N ′-Bis(2,6-dimethylphenyl)-3,4,9,10-perylenetetracarboxylic diimide. At the fixed temperature, the PM texture is dark ( Supplementary Fig. S3a ) as n̂ is perpendicular to the polarizer. Thermally induced flow in the direction perpendicular to the rubbing direction causes deviations of the director from the original state, seen as slight brightening of the PM texture ( Supplementary Fig. S3b ); the texture relaxes back to the original state when the temperature is stabilized ( Supplemenatry Fig. S3c) . The effect is more pronounced in the FCPM mode of observations that visualizes the vertical cross-section of the cell along the plane perpendicular to the rubbing direction ( Supplementary Fig. S3d,e,f ). As the polarization of the probing beam in FCPM is perpendicular to the rubbing direction, the states with a stable temperature are dark ( Supplementary Fig. S3d,f ), whereas the contraction-induced state is bright ( Supplementary Fig. S3e ). Supplementary Figure S4 shows the thermo-mechanical effect in a round quartz capillary (inner diameter 100 μm). The capillary was flashed with a weak solution of lecithin in hexane, to set the homeotropic alignment of n̂ (perpendicular to the capillary walls), and filled with E7. To minimize the elastic energy, n̂ realigns from the radial directions near the walls to an axial orientation in the center of capillary. This 'escaped' configuration often produces point defects at the axis, the so-called hedgehogs [21] (inset in Supplementary Fig. S4a ). As the temperature varies, NLC experiences transient flow, director reorientation, and displacement of hedgehogs ( Supplementary Movie 3 ). The experiments above clearly demonstrate the suitability of the effect for optofluidic applications, in which relatively small temperature variations cause dramatic optical changes. There are no fundamental obstacles for similar effects in other types of LCs, such as chiral (cholecteric) phases and smectic phases with partial positional order. High rates of temperature changes In the experiments above, the temperature was controlled by the hot stage with a relatively modest maximum rate ξ =0.5 °C s −1 . Much higher values of ξ can easily be achieved using electrodes, for example, transparent and conductive indium thin oxide. We verified that by applying the electric field (20 V, 1 kHz) to the indium thin oxide electrodes on the typical LC cells, one can increase ξ to (3–5) °C s −1 and flow velocities to about 100 μm s −1 . Transport of levitating colloidal particles Besides optofluidics, the described thermo-optical effect in LCs can also be used for a controlled transport of particles. In the nematic host, colloidal particles impose director distortions [22] . Elastic repulsion of these distortions from the bounding plates allows the particles to levitate in the NLC bulk [23] . This levitation effect is an important advantage of the LCs as compared with isotropic fluids in microfluidic applications, as it resists gravity and trapping of the particles at boundaries. The fluorescent latex spheres of diameter 2 μm used to trace the flows ( Fig. 1b ) in the expanding/shrinking slabs of NLC survive multiple thermal cycles, without being immobilized, remaining in the bulk of the material and resisting sedimentation. The most striking feature of the observed molecular realignment ( Fig. 4 ) is that the effect is caused simply by thermal expansion. The thermo-optical effect is uniquely attached to the orientational order and absence of the long-range positional order in the NLC. In a regular isotropic fluid, such an effect is impossible as there is no long-range orientational order. In a solid crystal, the effect is not possible because the changes in positional order are not sufficiently large to trigger molecular realignments. In a bounded NLC, the flow induced by thermal expansion and contraction is maximum in the central part of the sample but should vanish at the walls because of the no-slip conditions. The ensuing velocity gradients impose a reorienting torque on the director. Below we propose a simple analytical model of the observed thermo-mechanic and thermo-optical effects in the NLC. The mechanism of thermally induced flow is clear from the mass conservation equation [10] , which connects the time derivative of the fluid density ρ to the spatial gradients of its velocity. The density of a NLC slab thermally expanding or shrinking along its axis x can be presented as ρ ( t )= 0 (1− βξt ), where ρ 0 = ρ ( T = T 0 ) is the initial density of NLC. The mass conservation equation then immediately yields v x ∝ βξx , that is, a non-zero velocity along the axis x that depends linearly on the distance from the geometrical center x =0, rate ξ, and the coefficient β of thermal expansion. A more detailed consideration should take into account the boundary conditions and other (slower) components of velocity. The experimental conditions imply a low Reynolds number Re= ρdv x / |α 2 | ∼ 10 −6 , where |α 2 |=0.28 kg m −1 s −1 (ref. 24 ) is the anisotropic viscosity of E7 in the geometry under consideration [21] . Therefore, the velocity should satisfy the Stokes equation ∇ p=μ ∇ 2 v (here ∇ p is the pressure gradient and μ is the dynamic viscosity) [9] , as well as a no-slip condition v x =0 and no-penetration condition at the bounding walls. The solution for v x then follows as: The z component of flow velocity, is much smaller than v x at distances of interest, x ≫ d , 0< z < d . Here and in what follows, we neglect the small corrections β | ΔT |≤10 −2 as compared with 1 and assume that the velocity is not affected by the director orientation. The flow along the x axis realigns n̂ towards the x axis ( Figs 3f and 4 ). The viscous reorienting torque [8] , [21] is proportional to the shear rate ∂ v x / ∂ z that is vanishing at the walls and at the middle plane z = d /2, according to equation (1). The viscous torque is opposed by the elastic torque that tends to keep n̂ along the z axis; here K 3 is the Frank elastic constant of bend [8] . The balance of the two torques for small angles θ = θ ( z ) between n̂ and the vertical z axis determines the flow-induced director profile: The model is in good agreement with the experiments. First, v x in equation (1) increases with the rate ξ and with the coordinate x , being very close to the experimental data in Fig. 2a,b . For example, equation (1) predicts | v x |=13 μm s −1 at z = d / 2 and x =−22 mm if one uses the experimental data β ≈7.8×10 −4 per °C, ξ =0.5 °C s −1 , ΔT= 5 °C and d =50 μm. The measured velocities are 10 μm s −1 ( Fig. 2a,b ). The small difference is understandable because the particles tracers have a finite size and because they are located somewhat below the middle plane, as determined by FCPM. Second, the director profile, equation (2), is of the bow type, with n̂ remaining homeotropic at z =0; d / 2; d , and tilted in the regions 0 < z < d / 2 and d /2 < z < d , precisely as in Fig. 3f . Note that at the middle plane, z = d /2, the velocity is maximum, equation (1), but the velocity gradient and thus tilt, according to equation (2), are zero, as in the experiment ( Fig. 3b,d,f ). Using | α 2 |=0.28 kg m −1 s −1 , K 3 =1.95×10 −11 N (ref. 24 ), and d =50 μm in equation (2), one finds a significant tilt of n̂ , about 34° at z =0.2 d ; 0.8 d and x =−22 mm, sufficient to cause the bright birefringent states ( Fig. 1b ). The thermally induced flow produces a non-uniform director profile ( Fig. 3b,d,f ). The tilt angle θ ( z ) is negative in the top half of the sample and positive in the bottom part ( Fig. 3f ). When one tests the specimen with a technique such as polarizing microscopy, conoscopy, X-ray, and so on that probes a response integrated over the sample thickness, the thermo-optical effect can be confused with the formation of a biaxial NLC. The response integrated over the uniaxial NLC with the single local optical axis varying from point to point and the response from a genuine biaxial NLC with two optic axes defined in each point of the specimen and titled with respect to each other would be very similar to each other. Consider, for example, the split isogyres in the conoscopic patterns ( Figs 1b,c and 3b ) that are often considered as a signature of the biaxial NLC with two local optic axes with a non-zero angle Φ between them. The separation 2 a of the two isogyres is a quantitative measure [13] of where 2 R is the diameter of the field of view ( Fig. 1c ) NA is the numerical aperture of the microscope's objective, n̄ is the average refractive index of the NLC. A zero split (a Maltese cross pattern, see inset in Fig. 3a ) implies Φ=0 and a uniaxial character of the homeotropic NLC. However, if the director of the uniaxial NLC is not uniform, θ = θ ( z ), as in equation (2), then the isogyres would be also split, by a distance [14] , [25] where Inserting into equation (3) the values and θ( z )≠ const from equation (2), one finds that in a thermally expanding/shrinking uniaxial NLC the isogyres are split, with a separation that is proportional to the distance | x | from the center of capillary (as in the experiment, Fig. 1c ), cell thickness d , temperature change rate ξ and thermal expansion coefficient β . Therefore, the split isogyres are characteristic of not only a biaxial NLC but also of a uniaxial NLC that is thermally expanding or shrinking. Note that the phase diagrams of LCs are typically established by changing the temperature of the specimen; in these studies, one should be aware that thermal expansion/contraction of a uniaxial LC can mimic the appearance of biaxial states. The statement remains valid not only for conoscopic patterns but also for other techniques of characterization that measure an integrated response, such as polarizing microscopy, X-ray diffraction, and so on. Another important feature to bear in mind is that the temperature-triggered structural changes can be long lived, as suggested in Fig. 2c . Moreover, the director tilt might develop into the 'peak' structure [16] , [20] that is topologically distinct from the homeotropic state and can remain in a metastable state for a long time, requiring nucleation of disclination defects to relax back. The corresponding splitting of isogyres will be trapped as a long-lived metastable state. In conclusion, we demonstrated experimentally that temperature-induced density variations of NLC trigger flows that cause reorientation of molecules and optic axis ( Fig. 4 ). The physical mechanisms of coupled expansion, flow, flow-induced shear, resulting director reorientation and its optical features such as splitting of isogyres were explained by a simple model that agrees well with the experiments. To demonstrate the essence of phenomena, we focused on relatively well-studied materials such as E7. Even in this case, a modest rate of temperature changes ξ =±0.5 °C s −1 causes a director tilt by tens of degrees and flow velocities on the order of 10 μm s −1 ; velocities on the order of 100 μm s −1 are achieved in experiments with a higher ξ created by electric heating. In the future, it will be of interest to expand the studies of the thermal expansion-induced phenomena in LCs to the case when the source of heating is a focused laser beam. It would allow one to enrich the set of control parameters by adding the anisotropic thermophoretic effects (motion caused by a static thermal gradient, extensively explored for isotropic fluids [12] ) and reorienting torque resulting from coupling between the electric field of light and the director. The described thermo-optical and thermo-mechanical effects should be even more pronounced in LCs formed by molecules of a complex shape, for which thermal expansion is expected to be stronger than in E7. One example is a non-symmetrically substituted triazole abbreviated DT6Py6E6, with molecules of a pronounced bent-core shape, in which one can observe temperature expansion-triggered splitting of isogyres that mimics appearance of a biaxial nematic phase [26] . The thermo-optical phenomenon should be carefully accounted for in establishing the phase diagrams of LCs with phase transitions brought about by temperature changes, as the expansion/contraction of uniaxial states results in features mimicking those of biaxial phases. The NLC cells activated by unsteady temperature can be used for simultaneous thermo-mechanical and thermo-optical effects, such as transport of particles levitating in the NLC bulk with concomitant reorientation of optic axis around them. The simplicity of the observed phenomena that do not require pumps nor even electrodes to produce dramatic optical and mechanical changes suggests that they will find applications in a variety of fields, including sensors, photonics, lab-on-a-chip, micro- and optofluidics. NLC materials and capillaries We used rectangular capillaries of thickness d =50 μm, width w =1 mm and length 5 cm made of fused quartz (Fiber Optics Center). The capillaries were flashed with a weak solution of lecithin in hexane, to set the homeotropic alignment of n̂ , and filled with E7, which has the wide nematic range −62.5 °C ≤ T ≤ 60 °C. Thermally induced expansions/contractions were directed along the capillary axis x as the coefficient of volume expansion of fused quartz ( β ≈1.7×10 −6 per °C) is much lower than that of E7 ( β ≈7.8×10 −4 per °C at 25 °C, as measured in our laboratory). The temperature was controlled by a hot-stage LTS350 with a controller TMS94 (both Linkam Instruments) with 0.01 °C precision and a typical rate of temperature change ξ =±0.5 °C s −1 . Cooling was assisted by a circulation of liquid nitrogen. Fluorescent tracers of flow To trace the flow patterns, we added a small amount (<1 wt%) of fluorescently labelled polydivinylbenzene latex spheres of diameter 2 μm (Seragen Diagnostics, Inc.) to the NLC. The density of spheres ρ p =1.06×10 3 kg m −3 matched closely the density of E7 ρ E7 =1.03×10 3 kg m −3 (ref. 24 ) to prevent sedimentation. Sedimentation is also prevented by elastic levitation in the NLC bulk [23] . The three coordinates ( x , y , z ) of the particles were determined by FCPM [15] . The vertical optical slicing of the samples by FCPM showed that the latex beads levitated practically in the middle plane of the capillary, at z =(23±3) μm in capillaries of thickness d =50 μm. The trajectories of fluorescent tracers were analyzed with Image Pro 6.2 (Media Cybernetics) to extract the maximum velocity v x of particles along the x axis during the temperature change. Fluorescent anisometric dye In FCPM observations, the nematic mixture MLC-6815 (birefringence n ≈0.0517 at 25 °C and wavelength 550 nm) was doped with a tiny amount (0.01 wt%) of a fluorescent dye N,N′-Bis(2,6-dimethylphenyl)-3,4,9,10-perylenetetracarboxylic diimide (Sigma-Aldrich). The dye molecules are strongly elongated and align parallel to n̂ . How to cite this article: Kim, Y.-K. et al . Molecular reorientation of a nematic liquid crystal by thermal expansion. Nat. Commun. 3:1133 doi: 10.1038/ncomms2073 (2012).